High-rate lithiation-induced reactivation of mesoporous hollow spheres for long-lived lithium-ion batteries Mechanical and chemical degradations of high-capacity anodes, resulting from lithiation-induced stress accumulation, volume expansion and pulverization, and unstable solid–electrolyte interface formation, represent major mechanisms of capacity fading, limiting the lifetime of electrodes for lithium-ion batteries. Here we report that the mechanical degradation on cycling can be deliberately controlled to finely tune mesoporous structure of the metal oxide sphere and optimize stable solid–electrolyte interface by high-rate lithiation-induced reactivation. The reactivated Co 3 O 4 hollow sphere exhibits a reversible capacity above its theoretical value (924 mAh g −1 at 1.12 C), enhanced rate performance and a cycling stability without capacity fading after 7,000 cycles at a high rate of 5.62 C. In contrast to the conventional approach of mitigating mechanical degradation and capacity fading of anodes using nanostructured materials, high-rate lithiation-induced reactivation offers a new perspective in designing high-performance electrodes for long-lived lithium-ion batteries. High-energy density anodes for lithium-ion batteries, such as Si, Co 3 O 4 , Fe 3 O 4 and SnO 2 , typically suffer mechanical degradation resulting from lithiation-induced volume expansion, electrode pulverization and detachment from the conducting environment during long-term cycling, thus leading to a large irreversible capacity loss, low initial coulombic efficiency, and poor-rate capability and cycling stability [1] , [2] , [3] , [4] . The liquid electrolyte decomposes and forms a passivating solid–electrolyte interface (SEI) layer on the electrode surface during cycling, protecting the electrode from electrolyte solvent co-intercalation and preventing further decomposition of electrolyte [5] . The repetitive volume expansion/contraction during cycling can fracture the SEI layer and expose new active surfaces for SEI growth. A thicker SEI layer can form, consuming electrolytes and lithium ions, reducing electrical conductivity and retarding Li-ion diffusion. Therefore, chemical degradation associated with the side reaction between the electrode surface and electrolyte and the formation of unstable SEI can degrade battery performance tremendously [6] . Mechanical stress/strain and degradation on cycling can be mitigated by nanostructured electrodes such as nanoparticles (NPs) [7] , [8] , [9] , [10] , nanowires [3] , [11] , nanorods [12] , nanotubes [13] , [14] and nanofibres [15] , allowing enhancement of Li-ion diffusion, relaxation of inner lattice stress and reduction of electrode exfoliation, thus improving the cycling stability and rate performance, but they still suffer capacity degradation on prolonged cycling primarily due to the unstable SEI. To design a stable SEI at the interface between the electrolyte and electrode is crucial to achieve a stable and enhanced battery performance. Novel nanoarchitectured electrodes have recently been developed to tackle this issue, for example, hollow carbon nanotube-encapsulated Si NPs with empty space [16] and double-walled silicon nanotube [17] , exhibiting substantial improvement of cycling performance. However, the high surface area of nanostructured materials intrinsically leads to the formation of a large amount of SEI upon the decomposition of liquid electrolyte, and trapped lithium in the SEI layers results in a substantial first cycle irreversible capacity loss [18] . Hierarchically meso- and nanoporous hollow spheres are recognized as promising electrode materials for electrochemical energy storages [19] , [20] , [21] , [22] , [23] , [24] , and the unique structure provides an enhanced surface-to-volume ratio and reduced lengths for both mass and charge transports. The hollow sphere also provides extra space to mitigate volume expansion/extraction, thus displaying enhanced cycling stabilities, particularly at low current densities. In addition, micron- or submicron-sized hollow spheres assembled by nanosized particulates may show an ideal geometry for battery electrodes due to significantly less formation of SEI on the outer surface of the sphere as compared with larger surface area nanostructures. However, mesoporous hollow metal oxide spheres as electrodes still suffer severe mechanical degradation due to the drastic volume changes inherently accompanying with the conversion reaction and unstable SEI formation, leading to tremendous capacity fading as demonstrated in Co 3 O 4 nanospheres ( Fig. 1 ), particularly at high charge/discharge rates. 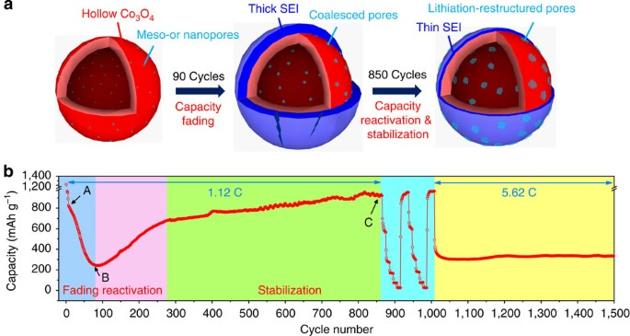Figure 1: Lithiation-induced reactivation. (a) Schematic evolution of mesoporous hollow spheres and SEI formation on long-term cycling. (b) The entire lithiation-induced reactivation process and cycling performance. Figure 1: Lithiation-induced reactivation. ( a ) Schematic evolution of mesoporous hollow spheres and SEI formation on long-term cycling. ( b ) The entire lithiation-induced reactivation process and cycling performance. Full size image Interestingly, beyond the capacity fading, high-rate lithiation-induced reactivation can occur for the hollow sphere metal oxide electrodes in which lithiation-induced mechanical degradation can effectively restructure the mesoporous hollow sphere and optimize a stable SEI layer. The reactivated electrode displays an excellent reversible capacity above its theoretical value and an unprecedented cycling stability without capacity fading even after an extremely long cycle at high rates. The process of reactivating electrode materials by high-rate lithiation is demonstrated in Fig. 1 consisting of three stages. Initial capacity fading occurs first due to mechanical degradation and unstable SEI formation on cycling, followed by capacity reactivation under continuous high-rate lithiation and eventually capacity stabilization. The high-rate lithiation-induced reactivation is due to a synergistic combination of the refinement of a hollow sphere into a hierarchically mesoporous structure and the optimization of stable SEI. Electrochemical reactions were previously demonstrated effectively in fabricating meso- and nanoporous structures with well-controlled pore structure and chemical compositions, greatly improving the performance of electrode materials [25] . Different mechanisms were proposed for the formation of porous structures, for example, by galvanic replacement reactions [26] due to different reduction potentials or through a nanoscale Kirkendall effect due to different diffusion rates of migrating species [27] , [28] , [29] . The lithiation-induced nanoporous structure formation typically occurs on metal, metal oxide and semiconductor nanocrystals/nanowires at initial lithiation/delithiation cycles (<10 cycles) [27] , [28] . By applying high-rate lithiation, the detrimental mechanical stress and large volume expansion can be deliberately controlled in refining porous architectures of the active materials and optimizing SEI formation to design long-lived battery electrodes. Using mesoporous Co 3 O 4 hollow spheres as an example, a new three-dimensional (3D) hierarchically mesoporous sphere consisting of an enlarged pore size/space and flower-like nanosheets can be created as a result of the constantly accumulative mesopores inside the active materials on cycling, accompanying with electrochemical reaction-induced solid state amorphization [30] . Concurrently, high mechanical stress by repetitive volume expansion of Co 3 O 4 and Li intercalation into the SEI layer [31] , [32] may fracture, exfoliate and reform thick SEI during the initial capacity fading period. With the structure refinement into more open mesoporous architecture by high-rate reactivation that can effectively buffer the volume expansion and mitigate stress impacting outward, a thin and stable SEI can be formed without fracture. Upon the high-rate lithiation reactivation, hierarchically mesoporous spheres display unique features for lithium-ion storage including a self-reconstructed open nanostructure with enlarged empty space withstanding repetitive volume changes, a nanoscale diffusion length of the active material allowing ultrafast mass and charge transports and a self-optimized thin and static SEI layer accommodating long-term cycling, enabling enhanced coulombic efficiency, exceptional rate capability and lifetime extension of battery materials. Lithiation-induced reactivation The hollow Co 3 O 4 spheres were synthesized by surfactant-assisted solvothermal decomposition of cobalt nitrate (a detailed procedure is given in the Methods) [33] , and the hollow and mesoporous sphere was verified by transmission electron microscopy (TEM) images and nitrogen adsorption–desorption isotherm measurements as shown in Supplementary Figs 1 and 2 , respectively. Despite the mesoporous and hollow structure of the metal oxide spheres, the capacity fading is tremendously ( Fig. 1b ) decreasing from 827 (at the second cycle) to 246 mAh g −1 (at the 90th cycle) at a current of 1.0 A g −1 (1.12 C, a rate of 1 C corresponding to complete charge or discharge in 1 h, 1 C=890 mAh g −1 ). The drastic capacity fading results from lithiation-induced mechanical degradation and the formation of unstable SEI. Amazingly, after capacity fading to the lowest value at the 90th cycle, continuous high-rate lithiation reactivates the electrode materials, increasing Li storage capacity monotonically during the subsequent cycles without signs of further degradation ( Fig. 1b ). The reactivated capacity can reach 783 mAh g −1 in the 500th cycle at 1.12 C, more than 300% capacity recovery from the lowest value at the same rate. A high reactivation capacity of 927 mAh g −1 after 850 cycles was achieved at 1.12 C, even higher than the initial capacity (the second cycle at the same rate). The significantly enhanced capacity is an ~250% improvement of the theoretical capacity of traditional graphite anode (~370 mAh g −1 ). The electrochemical properties such as coulombic efficiency, galvanostatic charge/discharge curves, cyclic voltammograms and Nyquist plots at different cycles were shown in Supplementary Figs 3–6 and Table 1 , and corresponding discussions. Coulombic efficiency of the electrode is 79.25% at the first cycle at 0.11 C (the first five cycles at 0.11 C and the following cycles at 1.12 C, Supplementary Fig. 3 ), and the large irreversible capacity loss is due to the formation of SEI layer [18] . At a rate of 1.12 C, it first increased to 98.53% at the 16th cycle, then decreased to 97.23% at the 49th cycle, followed by a gradual increase till the 110th cycle and finally stabilized at 99.83% afterwards. Note that coulombic efficiency ( Supplementary Fig. 3 ) is indicative of the stability of the SEI layer, closely relating to the lithiation-induced capacity degradation and reactivation ( Fig. 1b ). Nyquist plots ( Supplementary Fig. 6 ) and their corresponding kinetic properties ( Supplementary Fig. 7 and Table 1 ) indicate superior Li-ion diffusion and electron transport on lithiation-induced reactivation process. Lithiation-induced structure and morphology evolution High-rate lithiation-induced morphological and microstructure evolutions were investigated in detail on full charge/discharge at different cycles. The electrodes were decomposed in an argon dry box and residual electrolytes were removed by soaking electrodes in acetonitrile, then washed with ethanol and methanol, leaving inorganic SEI on the surface of electrode spheres. Ex situ X-ray diffraction (XRD) spectra (acquired 20 min each) are shown in Supplementary Fig. 8 , and the absence of diffraction peaks from crystalline Co 3 O 4 after being charged at 90 and 850 cycles suggests an electrochemical lithiation-induced crystalline to amorphous phase transition, consistent with the previous reports [28] , [30] . Meanwhile, the emerging diffraction peaks as observed in Supplementary Fig. 8 can be attributed to inorganic SEI layers including salts Li 2 CO 3 and Li 2 O. SEM images ( Fig. 2b,c ) show morphology of the pristine hollow spheres, demonstrating a rough surface in texture consisting of NPs. The SEI layers on various cycles are shown in SEM images ( Fig. 2d,h ) and TEM images ( Fig. 2e,i ) accordingly. Apparently, a thick SEI layer (~50 nm) formed (see TEM image in Fig. 2e ) and cracks as outlined inside the red dashed squares ( Fig. 2d ) are clearly visible in the thick SEI for electrode after 90 cycles (region B in Fig. 1b ). The longer diffusion length for lithium ions through the thicker SEI film, retarded electron transport as inferred from the Nyquist plots ( Supplementary Fig. 6 ) and the consumption of lithium ions and electrolyte during repetitive formation of SEI layers significantly degraded coulombic efficiency ( Supplementary Fig. 3 ) and cyclic stability of battery materials, as shown in the fading stage ( Fig. 1b ). In contrast, after 850 cycles (region C), a new thinner SEI layer (~15 nm thick, as shown in Fig. 2h,i ) evolved during the lithiation-induced reactivation process once the thicker SEI layer was exfoliated continuously due to the high surface stress [31] . This optimized thin SEI layer is generally stable against drastic volume change and fracture, contributing to the enhanced rate capability and long-lived cycling behaviour ( Fig. 1b ), consistent with the stable coulombic efficiency (as shown in Supplementary Fig. 3 ). 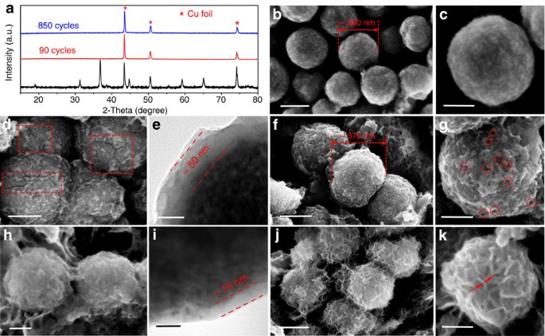Figure 2: Lithiation-induced structure and morphology evolutions. (a) XRD spectra of synthesized electrodes before and after 90 or 850 cycles at 1.12 C (the inorganic SEI was removed by washing in ethanol and methanol, then dipping in water for around 2 days), red stars representing the patterns from the Cu foil. (b,c) SEM images of synthesized electrodes before cycling. (d–g) SEM and TEM images of electrodes after 90 cycles at 1.12 C. The red dashed squares indindicate the cracks in the SEI layers, and the thick region of the non-uniform SEI layer as indicated by the red dashed lines ineis around 50 nm. SEM images inf,gshow the 90 cycled electrodes after inorganic SEI removal. The red dotted circles ingindicate the coalesced pores. (h–k) SEM and TEM images of electrodes after 850 cycles at the same rate. The thinner SEI layer inh,iis measured to be around 15 nm. SEM images inj,kshow the 850 cycled electrodes after inorganic SEI removal. The red arrows indicate the reduced diffusion length of flower-like nanosheets. Scale bar, 200 nm (b,d,f,j), 100 nm (c,g,h,k), 50 nm (e) and 20 nm (i). Figure 2: Lithiation-induced structure and morphology evolutions. ( a ) XRD spectra of synthesized electrodes before and after 90 or 850 cycles at 1.12 C (the inorganic SEI was removed by washing in ethanol and methanol, then dipping in water for around 2 days), red stars representing the patterns from the Cu foil. ( b , c ) SEM images of synthesized electrodes before cycling. ( d – g ) SEM and TEM images of electrodes after 90 cycles at 1.12 C. The red dashed squares in d indicate the cracks in the SEI layers, and the thick region of the non-uniform SEI layer as indicated by the red dashed lines in e is around 50 nm. SEM images in f , g show the 90 cycled electrodes after inorganic SEI removal. The red dotted circles in g indicate the coalesced pores. ( h – k ) SEM and TEM images of electrodes after 850 cycles at the same rate. The thinner SEI layer in h , i is measured to be around 15 nm. SEM images in j , k show the 850 cycled electrodes after inorganic SEI removal. The red arrows indicate the reduced diffusion length of flower-like nanosheets. Scale bar, 200 nm ( b , d , f , j ), 100 nm ( c , g , h , k ), 50 nm ( e ) and 20 nm ( i ). Full size image The decomposed electrode spheres were further treated to completely remove residual inorganic SEI by washing them in ethanol and methanol, then dipping in water for around 2 days [28] . The diffraction peaks of the inorganic SEI disappeared as shown in Fig. 2a , indicating that most of the inorganic salts like Li 2 CO 3 and Li 2 O were removed after washing process. After 90 cycles at 1.12 C (1.0 A g −1 ), the surface became rougher with an enlarged pore size (marked by red dashed circles in Fig. 2g ). Concurrently, an increase in the sphere size (~370 nm in diameter) was observed as compared with the original size of hollow spheres (~280 nm in diameter). The enlarged volume may probably be attributed to the lithiation-induced pore formation and coalescence inside of the spheres. Continuous high-rate lithiation refines the mesoporous hollow structure into a new 3D hierarchically mesoporous amorphous nanosphere consisting of enlarged pore size/space and flower-like nanosheets as shown in Fig. 2j,k . This morphological refinement is driven by the nanoscale Kirkendall effect between fast-diffusing cobalt in the cobalt nanograins and relatively slow-diffusing oxygen ions in the Li 2 O matrix [28] , [29] , [34] . Particularly, cobalt oxide anode material is based on the conversion reaction mechanism as follows: During the lithiation (discharge) process, 8Li can be inserted into Co 3 O 4 to form a Co/Li 2 O nanocomposite in which nanoscale Co clusters are embedded in the Li 2 O matrix, accompanied by a large volume expansion of active materials. When Li is extracted (during delithiation) out of the Co/Li 2 O nanocomposite, the expanded active materials contract in the charge process and end up with a volume larger than the original spheres, due to more free volume generated inside the material and the formation of mesopore in the hollow structure. The accumulation/enlargement of the pore structure essentially leads to the formation of the interconnected flower-like nanosheets with the thickness of only a few nanometres, as indicated by the red arrows in Fig. 2k , favourable for fast transport of lithium ions and electrons. The detailed mechanism for the stable SEI on high-rate lithiation and reactivation is elaborated in the schematic in Supplementary Fig. 9 . Before reactivation, mesoporous hollow spheres can buffer the volume changes to some extent at low rates and initial cycles. Under a high-rate charge/discharge and longer cycles, the mesoporous hollow spheres suffer high mechanical stress due to the large and repetitive volume expansion/contraction of Co 3 O 4 . The outside SEI layer may fracture, exfoliate and reform leading to the unstable and thick SEI ( Fig. 2d,e ). The consumption of Li and thick SEI layer formation in slowing down Li-ion transport behaviour greatly degrade the electrochemical performance. After reactivation, the refined more open mesoporous structure with interconnected nanoscale sheets and larger free volume inside gradually form, offering a more favourable way for the inward volume change in the internal structure during full lithiation process, and it may gradually convert back to the original architecture during delithiation process. Thus, the reactivated hierarchical mesoporous structure is becoming more robust against repetitive volume changes, and its outside SEI layer is subjected to much less mechanical stress induced by volume changes and are more stable without fracture ( Fig. 2h,i ). Therefore, the inside robust lithiation-tailored unique nanostructure of active materials and the outside optimized static and thin SEI layers lead to a dramatically reactivated lithium storage capacity, an improved coulombic efficiency and long-lived and stable cycling performance ( Fig. 1b ; Supplementary Fig. 3 ). Rate capability and cycle performance after reactivation High-rate lithiation-reactivated electrode also exhibits greatly enhanced rate capability. 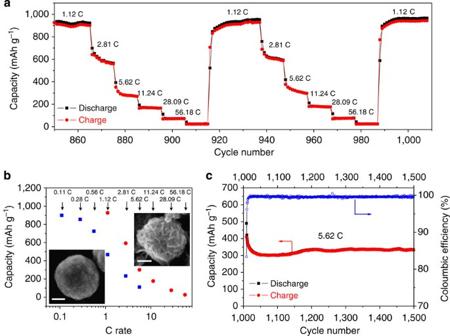Figure 3: Electrochemical performance of the Co3O4after high C-rate reactivation process. (a) Cycling performance at various rates from 1.12 to 56.18 C after 850 cycling at 1.12 C. (b) The comparison of rate capability before and after lithiation-induced reactivation. Blue squares and red circles indicate the average capacity at each rate before and after reactivation, respectively. Scale bar, 100 nm. (c) Capacity retention and coulombic efficiency at a higher rate of 5.62 C for the subsequent 500 cycles after 1,000-cycling test. Figure 3a is the close-up of twice successive sequence tests at various rates from 1.12 C (1.0 A g −1 ) to 56.18 C (50 A g −1 ) following the capacity fading, reactivation and stabilization stages shown in Fig. 1b . The reactivated electrode can deliver a stable capacity of 929 mAh g −1 at 1.12 C, 610 mAh g −1 at 2.81 C, 321 mAh g −1 at 5.62 C, 181 mAh g −1 at 11.24 C, 76 mAh g −1 at 28.09 C and 26 mAh g −1 at 56.18 C. More importantly, the reversible capacity of the electrode can recover to its initial capacity value of 934 mAh g −1 at 1.12 C after twice successive sequence measurements. Figure 3b compares the corresponding capacities of the sequence tests before (blue squares, the sequence test of inactivated electrode shown in Supplementary Fig. 10 ) and after reactivation (red circles). Obviously, significantly enhanced rate capability was demonstrated on lithiation-induced reactivation. For instance, the reversible capacity at a rate of 1.12 C after reactivation is 200% greater than that before the reactivation at the same rate, and even higher than that at lower rates of 0.11–0.56 C before reactivation. The reactivated electrode also exhibits a remarkable cyclic stability for lithium storage at a higher C rate of 5.62 C (5.0 A g −1 ) for the subsequent 500 cycles that followed the previous 850 cycling and twice successive sequences ( Fig. 3c ). Stable reversible capacity and coulombic efficiency were observed during the whole 500 cycles and the capacity stabilizes at 335 mAh g −1 , almost a 300% capacity improvement as compared with electrodes without reactivation. Figure 3: Electrochemical performance of the Co 3 O 4 after high C-rate reactivation process. ( a ) Cycling performance at various rates from 1.12 to 56.18 C after 850 cycling at 1.12 C. ( b ) The comparison of rate capability before and after lithiation-induced reactivation. Blue squares and red circles indicate the average capacity at each rate before and after reactivation, respectively. Scale bar, 100 nm. ( c ) Capacity retention and coulombic efficiency at a higher rate of 5.62 C for the subsequent 500 cycles after 1,000-cycling test. Full size image Varying reactivation schemes via controllable C rates The capacity fading and reactivation processes of the mesoporous hollow spheres are affected significantly by different charge/discharge (D–C) rates. The reactivation capacity can be finely tuned by controlling mechanical stress associated with lithiation/delithiation processes and thus microstructure evolutions at different D–C rates. To further understand the effects of lithiation/delithiation and shorten the cycling time on the process of capacity fading and reactivation, different schemes of D–C rates were tested: (1) constant D–C rates (as shown in Fig. 4a with different rates of 0.45, 1.12, 1.69 and 2.81 C to 500 cycles and also denoted as CC rate by the black curve in Fig. 4b ); (2) varied D–C rates (denoted as VC rate by the red curve in Fig. 4b ) with a higher D–C rate of 2.81 C (2.5 A g −1 ) for the capacity fading till 90 cycles and a relatively lower D–C rate of 1.69 C (1.5 A g −1 ) for capacity reactivation till 265 cycles; and (3) mixed D–C rates (denoted as MC rate by the blue curve in Fig. 4b ) with a higher discharge rate of 2.81 C and a relatively lower charge rate of 1.69 C in each cycle for the capacity fading and reactivation stages up to 400 cycles. A high D–C rate of 2.81 C was performed afterward for each scheme after reactivation to test the long-lived cyclic stability of the reactivated electrodes. 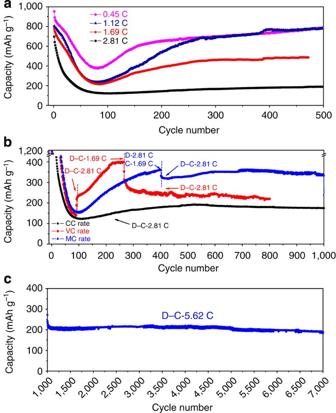Figure 4: Varying reactivation schemes via controllable C rate. (a) The capacity retention of the as-prepared anode at a constant rate of 0.45, 1.12, 1.69 or 2.81 C. (b) Comparison of various C-rate schemes for lithiation-induced reactivation process. (c) Long cycling performance at a high rate of 5.62 C after MC-rate reactivation process. Figure 4: Varying reactivation schemes via controllable C rate. ( a ) The capacity retention of the as-prepared anode at a constant rate of 0.45, 1.12, 1.69 or 2.81 C. ( b ) Comparison of various C-rate schemes for lithiation-induced reactivation process. ( c ) Long cycling performance at a high rate of 5.62 C after MC-rate reactivation process. Full size image The drastic impacts of D–C rates on the capacity fading and reactivation can be summarized as follows. First, electrodes at higher D–C rates suffer more capacity fading in general, and can be reactivated to a less reversible capacity. For example, very limited reactivation capacity was achieved at 2.81 C (189 mAh g −1 ), and the maximum reactivation capacity was delivered at 1.12 C (783 mAh g −1 ) shown in Fig. 4a . Therefore, an optimized lithiation rate, for example, 1.12 C, can be identified to achieve highly reactivated capacity and rate performance. At a lower C rate of 0.45 C, electrodes experience less capacity fading and thus less capacity reactivation, and the capacity achieved is similar to that of 1.12 C (see Fig. 4a ). The reactivation can be completed at ~150 cycles. The various high-rate performance of electrodes after 500-cycle reactivation at both high (1.12 C) and relatively low rates (0.45 C) was compared in Supplementary Fig. 11 . Although capacities were reactivated at the same level by different rates after 500 cycles, the electrode materials on 1.12 C reactivation can deliver better electrochemical performance at high rates than that on low-rate reactivation (0.45 C). At the optimized charge/discharge rate (1.12 C) for reactivation, vigorous mechanical stress and fast volume changes can efficiently refine the morphology and structure of the mesoporous electrodes, thus fully reactivating electrodes to enhance performance at higher C rates. As compared with the mesoporous hollow spheres, no capacity reactivation occurs in solid Co 3 O 4 NPs with the size of ~30 nm as a control sample ( Supplementary Fig. 12 ). As the vigorous volume changes under high C-rate lithiation is necessary for the reactivation process, for solid Co 3 O 4 NPs, pulverization instead of reactivation may occur. The large irreversible capacity loss without reactivation for solid Co 3 O 4 NPs may also be associated with the significant formation of unstable/thicker SEI as a result of large surface area of the small-sized particles, consistent with the degraded Li-ion diffusion kinetic and increased surface film and charge transfer resistances as indicated in Supplementary Fig. 13 . Therefore, the mesoporous hierarchically hollow spheres show an ideal geometry for capacity reactivation: intrinsically free space and hollow geometry in mitigating volume changes without pulverization, and the relatively large size (sub-microns) in a spherical geometry reducing the amount of SEI formation on the outer surface of the spheres as compared with large surface area NPs. Second, the lithiation/delithiation rates at the capacity reactivation stage dominate the capacity recovery and electrode cyclic stability. For instance, the electrodes charged at a constant rate of 1.69 C (red curve in Fig. 4a ) delivered almost the same reactivated capacity (~420 mAh g −1 ) as they charged at the VC rate of 1.69 C (red curve in Fig. 4b ) for the reactivation despite that a greater D–C rate (2.81 C) for the capacity fading stage. These results indicate that the mechanical degradation during the capacity fading stage does not significantly affect the capacity reactivation of electrode. In addition, electrodes reactivated at lower D–C rates displayed a greater capacity (as inferred by comparing VC-rate and CC-rate schemes cycled at the same D–C rate of 2.81 C after different rates for reactivation). Finally, the scheme of controllable lithiation (discharge)/delithiation (charge) rates at the capacity fading and reactivation stages plays a pivotal role in determining the performance of reactivated electrodes. The electrode reactivated with the MC rate (a higher discharge (lithiation) rate and a lower charge (delithiation) rate for each cycle) exhibited a significantly higher reversible capacity (345 mAh g −1 ) than those reactivated with VC rate (223 mAh g −1 ) or CC rate (189 mAh g −1 ) under the same high D–C rate of 2.81 C. A greater discharge rate will lead to higher mechanical stress and thus a fast volume expansion on the Li-ion insertion into active materials (lithiation process) to form metal/Li 2 O nanocomposites. During the delithiation process, a slower atomic diffusion is expected as driven at a lower charge rate, leading to more efficient formation of nanoscale pores and refinement of the mesoporous structure [28] . The more significant mechanical stress, vigorous volume change and efficient pore formation during the fast lithiation and slow delithiation processes may favour greater morphological and structural refinements and rescaling of the porous structure at a smaller scale, significantly improving the lithium storage performance at high rates. This reactivated electrodes also display remarkable long cycling performance charged at high C rates. For the electrode reactivated with the 400-cycle MC-rate scheme, the reversible capacity was retained at 345 mAh g −1 at 2.81 C for the next 600 cycles and 219 mAh g −1 at 5.62 C for the subsequent 6,000 cycles without a sign of performance degradation ( Fig. 4c ). Mass loadings on lithiation-induced capacity reactivation High mass loadings of active materials are more desirable for commercial applications to achieve high volumetric energy density. In general, the electrochemical performances of electrodes are degraded at high mass loadings. The effects of mass loading on high-rate capacity reactivation of the mesoporous hollow electrode were tested at a rate of 1.12 C, as shown in Supplementary Fig. 14 . A high capacity and stable cycling performance at an increased areal mass loading of 1.7 mg cm −2 can be maintained. At higher mass loadings of 2.3 and 2.8 mg cm −2 , the reactivated capacities stabilize at 650 and 370 mAh g −1 , respectively. It is expected that longer cycles are needed to fully reactivate electrodes due to more active materials, and slower transport behaviour at greater mass loadings may also affect the reactivation efficiency. As compared with graphite anode, the commercial anode materials for lithium-ion batteries, the reactivated electrodes show superior performance (at least 600–800% enhancement) when charged at the same rate and comparable mass loadings (for example, 1.6 and 2.6 mg cm −2 ), as shown in Supplementary Fig. 14 . Note that the current tests were performed on a coin cell configuration, and an enhanced efficiency of reactivation is expected at greater mass loadings in commercial pouch or cylinder cell configurations. To achieve similar volumetric energy density as commercial LIB using graphite as anode, less mass loading is required for the reactivated electrode due to greatly enhanced capacity with simultaneously enhanced cyclic stability and power density. Note that the strategy of using high C-rate lithiation to reactivate electrodes by tailoring microstructure and optimizing SEI formations is in contrast to the routine practice of the industry using low C-rate pre-lithiation to develop a stable SEI layer and activate electrode of battery systems. Ideally, greater D–C rates are desired for practical applications by our high C-rate lithiation method, allowing completion of rapid capacity fading and reactivation. A trade-off is expected between short reactivation time (high C rate) and high lithium storage performance. The MC-rate scheme (D-2.81 C and C-1.69 C) enables the electrode reactivation within 3.5 days to 400 cycles, and the reactivated materials offer tremendous potentials used as advanced electrodes in long-lived lithium-ion battery systems with unprecedented cycling stability and high-rate performance. Here we further demonstrate a proof of concept that the high-rate pre-lithiation and reactivation can be applied to first restructure active materials and optimize SEI ex situ to obtain high-performance electrodes. After pre-lithiation and pre-reactivation, the electrode materials with optimized microstructure can be packaged into battery cells for practical applications with exceptional rate performance and cyclic stability. Pre-lithiation method is typically utilized for Li-free cathode materials, such as V 2 O 5 (ref. 35 ), MoO 3 (ref. 36 ) and sulphur [37] , to improve their energy density. In this study, pre-lithiation and pre-reactivation of our anode materials were conducted by a self-designed open-cell geometry (see Supplementary Fig. 15 and Methods) in a glove box, in which the lithium metal can be used as the counter electrode to provide an unexhausted source of lithium for pre-lithiation purpose. Similar to in situ lithiation and reactivation in a half-cell ( Fig. 1b ), the capacity fading and reactivation were also observed for the open-cell configuration. After pre-lithiation and reactivation processes for 400 cycles at 1.4 C, the electrode materials and a new lithium foil were assembled into a normal coin cell displaying exceptional performance with the first cycle coulombic efficiency of 98.7% and a continuously improved capacity at a rate of 1.4 C, as shown in Supplementary Fig. 16 . This is in a sharp contrast to the first cycle coulombic efficiency of 79.25% for electrode without pre-lithiation. No noticeable first cycle irreversible capacity loss is a result of stable SEI formation during the pre-lithiation process. The optimized microstructure and stable SEI during the pre-lithiation process enable highly stable electrodes without any chemical and mechanical degradations, and no capacity decay occurs at longer cycles and high C rate. Therefore, by refining and optimizing microstructure/forming stable SEI first through pre-lithiation and pre-reactivation, the reactivated electrodes show immense potentials for practical applications. In summary, we have demonstrated that the mechanical degradation on cycling can be deliberately controlled to finely tune mesoporous structure of the metal oxide hollow sphere and optimize stable SEI by high-rate lithiation-induced reactivation. The reactivated Co 3 O 4 hollow sphere exhibits a high reversible capacity above its theoretical value, enhanced rate performance and a cycling stability without capacity fading after 7,000 cycles at high rates. In contrast to the conventional approach of mitigating mechanical degradation and capacity fading of anodes using nanostructured materials, high-rate lithiation-induced reactivation offers a new perspective in designing high-performance electrodes for long-lived lithium-ion batteries. The strategy of high-rate lithiation-induced restruction and SEI optimization may also be applied to activate other metal oxides, sulphides, seleniums, fluorides, chlorides, nitrides and phosphides [34] , [38] , [39] , [40] , [41] , [42] , [43] , in which hierarchically porous structure can be produced with the same mechanism. Synthesis of electrode material The hollow and mesoporous Co 3 O 4 spheres were synthesized using a surfactant-assisted solvothermal method [33] . Specifically, 2.4 mmol of Co(NO 3 ) 2 ·6H 2 O and 0.8 ml of deionized water were dissolved in 22 ml of absolute methanol to form a red solution. Next, 5.7 mmol of sodium dodecylbenzenesulphonate was added to the solution in an ultrasonic bath for 30 min to form a suspension. Subsequently, the suspension was sealed in a 50-ml Teflon-lined autoclave and maintained at 200 °C for 4 h. After the suspension was naturally cooled to room temperature, the precipitates were collected and washed with deionized water and ethanol ultrasonically and then separated by centrifuging. The precipitates were vacuum dried at 90 °C for 2 h for subsequent experiments. Material characterizations XRD was performed using a PANanalytical XRD system with Cu source (wavelength of 1.542 Å) at room temperature. The surface area of Co 3 O 4 anode material was measured by a Quantachrome Autosorb-1 instrument. The morphology and microstructure of materials were characterized by a Carl Zeiss Supra field-emission scanning electron microscopy and a JEOL 2010 TEM operated at 200 keV. Cell preparation and electrochemical measurements The working electrodes were prepared by mixing 80 wt% active materials (Co 3 O 4 ), 10 wt% acetylene black (super-Li) and 10 wt% polyvinylidene fluoride binder dissolved in N -methyl-2-pyrrolidinone. After the above mixture was coated on Cu foils, electrodes were dried at 120 °C under vacuum for 12 h to remove the solvent, and then punched into a disk and pressed. The mass loading of the electrode material is between 1.0 and 2.8 mg cm −2 . Electrochemical measurements were performed using two-electrode CR 2032 coin-type cells with lithium foil as the counter electrode, Celgard 2340 membrane separator and 1 M LiPF 6 electrolyte solution dissolved in a 1:1 (v/v) mixture of ethylene carbonate and dimethyl carbonate. The cells were assembled in an argon-filled glove box with both moisture and oxygen contents below 1.0 p.p.m. Galvanostatic charge–discharge cycles were tested with the use of an Arbin Instrument at various rates of 0.11–56.18 C (0.1–50.0 A g −1 ) and a voltage window of 0.01–3.00 V. Cyclic voltametry (0.01–3.00 V, 0.5 mV s −1 ) and electrochemical impedance spectroscopy (0.1 Hz–100 kHz, 10 mV) were measured by an electrochemical workstation (Ametek, Princeton Applied Research, Versa STAT 4) at room temperature. Pre-lithiation and pre-reactivation The pre-lithiation was carried out for repetitive charge/discharge cycles at a rate of 1.4 C by a self-designed open-cell set-up ( Supplementary Fig. 15 ) in the glove box (both moisture and oxygen contents below 1.0 p.p.m.). Celgard 2340 membrane separators were used to separate two electrodes and prevent shorting (one between two electrodes function as normal separator, the other prevent shorting). The same electrolyte was dropped on the separators and electrodes. Copper stripes were used to connect the lithium metal and anode to an Arbin battery station to monitor pre-lithiation process. After pre-lithiation and reactivation in an open-cell test, the same electrode was packaged into a normal coin cell battery for electrochemical performance evaluation. How to cite this article : Sun, H. et al. High-rate lithiation-induced reactivation of mesoporous hollow spheres for long-lived lithium-ion batteries. Nat. Commun. 5:4526 doi: 10.1038/ncomms5526 (2014).